The impact of agricultural emergence on the genetic history of African rainforest hunter-gatherers and agriculturalists The emergence of agriculture in West-Central Africa approximately 5,000 years ago, profoundly modified the cultural landscape and mode of subsistence of most sub-Saharan populations. How this major innovation has had an impact on the genetic history of rainforest hunter-gatherers—historically referred to as ‘pygmies’—and agriculturalists, however, remains poorly understood. Here we report genome-wide SNP data from these populations located west-to-east of the equatorial rainforest. We find that hunter-gathering populations present up to 50% of farmer genomic ancestry, and that substantial admixture began only within the last 1,000 years. Furthermore, we show that the historical population sizes characterizing these communities already differed before the introduction of agriculture. Our results suggest that the first socio-economic interactions between rainforest hunter-gatherers and farmers introduced by the spread of farming were not accompanied by immediate, extensive genetic exchanges and occurred on a backdrop of two groups already differentiated by their specialization in two ecotopes with differing carrying capacities. The transition from hunting and gathering to farming was a major cultural innovation that spread over most of the globe during the last 10,000 years [1] . In sub-Saharan Africa, there is evidence coming from multidisciplinary approaches to indicate that agricultural technologies emerged ca . 5,000 years before present (YBP), in the area that corresponds today to Southeast Nigeria and Western Cameroon [2] , [3] . Early farming societies subsequently expanded from this region to much of Eastern, Central and Southern Africa, concomitantly with the diffusion of Bantu languages [4] , [5] , [6] . Most sub-Saharan populations adopted the agricultural, sedentary lifestyle associated with the expansions of Bantu-speaking peoples. However, a few groups, such as the hunter-gatherers inhabiting the Central African rainforest, the San from Southern Africa, or the Hadza and Sandawe from Eastern Africa, have continued to live as mobile bands, maintaining a mode of subsistence based primarily on hunting and gathering, although some of these groups have recently settled in villages. A major open question concerns how the emergence and spread of agricultural-related technologies have had an impact on the population dynamics and demographic history of African hunter-gatherers and farmers over time. In this context, the Central African belt, which is adjacent to the postulated homeland of Bantu-speaking peoples [3] , [4] , [5] , [6] , represents a key region to tackle this question, as the largest group of African hunter-gatherers, the rainforest hunter-gatherers (RHG—collectively known by the historical term ‘pygmies’, often locally used derogatively), coexist in this region with well-established agriculturalist (AGR) communities. Nowadays, RHG populations are subdivided into two main groups reflecting their geographic location, the ‘Western RHG’ and the ‘Eastern RHG’, each including multiple distinct populations [7] , [8] . In addition to a forest-dwelling mode of subsistence, both groups share distinctive cultural and phenotypic traits, such as specific hunting and honey-gathering techniques [9] , [10] and a reduced stature [11] , [12] , [13] . Archaeological and linguistic evidence indicate that the Central African rainforest has been densely peopled for more than 40,000 years [14] and that the first farmers settled across a vast expanse of this territory as early as 3,000–5,000 YBP [2] , [3] , [15] , [16] , [17] . As soon as farming communities penetrated the rainforest, extensive economic and technological exchange with local hunter-gatherers occurred, as attested by the appearance of pottery and polished stone tools within this time frame, together with the shared language families and oral traditions of the two communities [2] , [3] , [7] , [8] , [11] , [15] , [16] , [17] , [18] , [19] . Such early interactions are further supported by a recent study that reports the acquisition of Helicobacter pylori bacteria strains by Western RHG through contacts with their AGR neighbours ~4,500 YBP [20] . However, whether such interactions, especially during the earliest phases of the farmers’ settlement, triggered extensive gene flow between the two groups remains to be elucidated. Similarly, little is known about whether the signals of reduced effective population size currently observed in RHG [21] , [22] , [23] , [24] , [25] result from recent bottlenecks occurring in the last millennia, highlighting the impact of the expansion of Bantu-speaking farmers in fragmenting these populations, or from more ancient events possibly linked to their forest-dwelling lifestyle. Recent genome-wide studies based on single nucleotide polymorphism (SNP) array data or whole-genome sequences have documented the somewhat genetic isolation of RHG and identified candidate genes involved in their relatively small stature as well as other adaptive traits [22] , [26] , [27] , [28] . However, these reports were based on a single or small number of RHG populations, or focused on a limited geographic area (that is, West-Central Africa), despite the fact that they occupy a vast territory extending west-to-east in the equatorial rainforest from the Congo Basin to Lake Victoria. A detailed genome-wide picture of both the patterns of substructure among the different RHG groups and the degree of admixture between these populations and neighbouring AGR is thus missing. Here we present a high-resolution study of the genomic diversity of and relationships between both Western and Eastern RHG and neighbouring AGR populations, with the aim of dissecting the intensity and tempo of the admixture processes and demographic events that have characterized the past history of these human groups. We find that extensive admixture between the RHG and AGR groups has occurred only recently, within the past ~1,000 years, indicating that the early expansions of Bantu-speaking people did not trigger immediate, extensive genetic exchange between two communities. Furthermore, our results support the hypothesis that the ancestors of these two populations already differed in their demographic success before the emergence of a farming-based lifestyle in Central Africa. 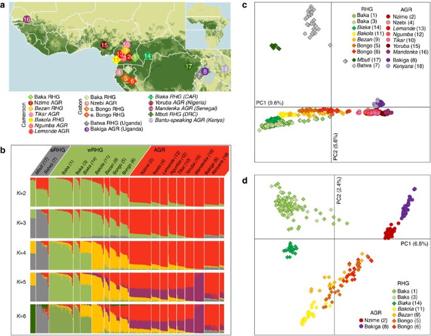Figure 1: Genome-wide structure of RHG and AGR populations. (a) Geographic locations of African populations studied here, including the RHG and AGR populations of this study and a selection of populations (in italics) retrieved from previous studies26,29. (b) Admixture analysis of 310,883 SNPs in 481 sub-Saharan Africans. Each vertical line is an individual. The colours represent the proportion of inferred ancestry fromKancestral populations. The minimal cross-validation error was observed forK=3. (c) PC analysis of 310,883 SNPs in 481 sub-Saharan Africans. PC1 and PC2 are presented with the proportion of variance explained. (d) PC analysis of 308,771 SNPs in 302 individuals from Western RHG and AGR populations. Numbers in brackets inb–dcorrespond to the population locations represented ina. Population genome-wide data set We generated genome-wide data from a collection of ethnologically well-defined populations of RHG and AGR, specifically chosen to study admixture processes ( Supplementary Table 1 ). These populations include Western RHG (Baka of Gabon, Baka of Cameroon, Bongo of South and East Gabon), Eastern RHG (Batwa of Uganda) and AGR neighbouring populations (Nzime, Nzebi and Bakiga; Fig. 1a ). We genotyped 1,048,713 SNPs in 327 individuals using the Illumina HumanOmni1 SNP array. In total, 930,134 autosomal and X-linked SNPs passed quality control filters, and 32 individuals were discarded owing to low call rates, Mendelian inconsistencies among trios and cryptic relatedness (Methods; Supplementary Fig. 1 ). Ultimately, 295 individuals were retained for subsequent analyses, including 216 unrelated individuals, 21 complete trios and 8 duos, totalling 266 unrelated samples. This data set was analysed in conjunction with genome-wide data from 11 additional African populations [26] , [29] , including 4 Western RHG populations (Baka, Bakola and Bezan of Cameroon, and Biaka of Central African Republic—CAR), 1 Eastern RHG population (Mbuti of the Democratic Republic of Congo) and 6 AGR relevant populations ( Fig. 1a ; Supplementary Table 1 ). Figure 1: Genome-wide structure of RHG and AGR populations. ( a ) Geographic locations of African populations studied here, including the RHG and AGR populations of this study and a selection of populations (in italics) retrieved from previous studies [26] , [29] . ( b ) Admixture analysis of 310,883 SNPs in 481 sub-Saharan Africans. Each vertical line is an individual. The colours represent the proportion of inferred ancestry from K ancestral populations. The minimal cross-validation error was observed for K =3. ( c ) PC analysis of 310,883 SNPs in 481 sub-Saharan Africans. PC1 and PC2 are presented with the proportion of variance explained. ( d ) PC analysis of 308,771 SNPs in 302 individuals from Western RHG and AGR populations. Numbers in brackets in b – d correspond to the population locations represented in a . Full size image Genetic structure of RHG and AGR populations To gain global insights into the population structure of RHG and AGR, we used the unsupervised clustering algorithm Admixture [30] and the principal component (PC) analysis implemented in EIGENSTRAT [31] . Clusters at K =2 and PC1 broadly separated RHG (both Western and Eastern) from AGR, and clusters at K =3 and PC2 then distinguished Western and Eastern RHG ( Fig. 1b,c ; Supplementary Figs 2–4 ). These observations are consistent with the proposed branching model of these populations—based on a limited number of autosomal and uniparentally inherited markers—involving an early divergence of the ancestors of RHG and AGR ~50,000–65,000 YBP, followed by a split of RHG ancestors into the Western and Eastern groups ~20,000–30,000 YBP [21] , [23] , [24] , [25] , [32] . The levels of genetic differentiation among RHG populations generally followed the isolation-by-distance model (Mantel’s test P =0.002), with the Batwa and Mbuti Eastern RHG representing, however, a clear exception to this model ( Fig. 1b,c ; Supplementary Fig. 5 ). 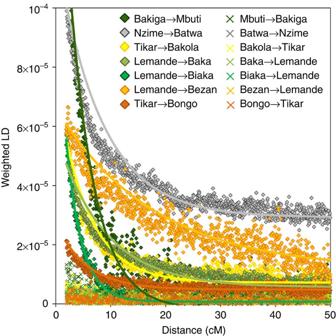Figure 2: Admixture LD in RHG and AGR populations. Admixture LD signals were detected with ALDER, using the one-reference mode with 363,088 SNPs in 481 sub-Saharan Africans. Lines represent fitted exponential curves for significant AGR-to-RHG admixture signals. Results for all possible pairs are reported inSupplementary Table 4. The AGR and RHG pairs plotted here correspond to populations that are known to interact today. If the corresponding AGR population was not sampled, or if a long-range LD correlation was observed between the two populations, the genetically closest AGR population was selected. Indeed, the Batwa and the Mbuti presented substantial levels of population differentiation ( F ST =0.036, Supplementary Table 2 ) despite their relatively close geographic proximity (~400 km). This degree of differentiation is comparable to that observed between Western and Eastern RHG groups ( F ST =0.038), which are separated by more than 1,500 km, suggesting unexpectedly strong genetic isolation among Eastern RHG ( Supplementary Note 1 , Supplementary Fig. 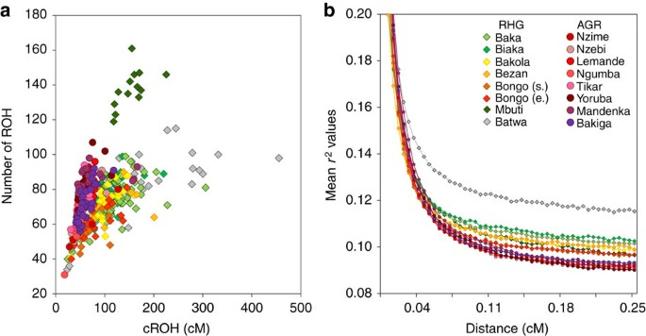Figure 3: Lower effective population sizes of RHG with respect to AGR populations. (a) Patterns of runs of homozygosity (ROH) in RHG and AGR populations. Cumulative ROH (cROH) is reported per population, against the total number of observed ROH. Population colour codes are reported inb. (b) LD decay with genetic distance in RHG and AGR populations. Pairwiser2values were obtained using Haploview, calculated between ~350,000 SNPs with minor allele frequency>5% in each population and averaged across 10 random samplings of 13 samples per population. On average, ~28 million values were obtained per population. 6 , Supplementary Table 3 ). This contrasts with the patterns observed among Western RHG populations where weaker genetic differentiation was observed ( F ST =0.014). Some population substructure was nevertheless detected in Western RHG who clustered into three distinct groups: the Baka of Cameroon and Gabon, the Biaka of CAR and a group composed of the Bakola and the Bezan of Cameroon and the Bongo of Gabon ( Fig. 1d ). Interestingly, the closest population to the Baka RHG—the only group of Western RHG speaking a non-Bantu Ubangian language—were the Bantu-speaking Biaka RHG of CAR ( F ST =0.010, Supplementary Table 2 ), with whom they share specific lexica related to the forest and hunting and gathering techniques [9] , [33] . Our analyses ( Supplementary Fig. 5 ), together with linguistic data, support the hypothesis that the Baka and Biaka Western RHG separated recently and that, although they adopted different AGR languages, they continued to use terms from an ancestral, extinct *Baakaa language [9] , [33] . Substantial degree of AGR ancestry in most RHG populations Despite the overall genetic distinctiveness of RHG and AGR populations, our data revealed that a substantial number of RHG individuals, both Western and Eastern, show high proportions of AGR ancestry, up to 68.6% ( Fig. 1b ; Table 1 ). Nevertheless, AGR ancestry proportions differed among RHG populations: while the mean was lower than 6% in Mbuti Eastern and Biaka Western RHG, it reached 38.5 and 47.5% in Bezan and Bongo Western RHG, consistent with the higher stature and social integration in agricultural communities of the latter groups [25] , [34] , [35] . Conversely, the proportions of RHG ancestry among all AGR individuals were systematically low, ranging from 0.7 to 15.7% with a mean of 10.2%. These observations suggest either the occurrence of asymmetrical gene flow from AGR to most RHG populations or symmetrical gene flow between populations differing in their effective population size. Table 1 Proportions of RHG and AGR ancestry among African populations. Full size table We next formally tested for the occurrence of admixture between RHG and AGR, using the extent of admixture linkage disequilibrium (LD) [36] . This approach, implemented in ALDER [37] , was applied to all possible pairs of populations, including a test population and a single surrogate parental population. Tests based on two parental populations were not considered here, as there is no RHG population that can be used as a truly non-admixed reference. Our analyses showed that signals of AGR-to-RHG admixture were clearly significant in all RHG populations and involved admixture rates of at least 15%, while those of RHG-to-AGR admixture were either non-significant or yielded admixture rates lower than 4%, in all AGR populations ( Fig. 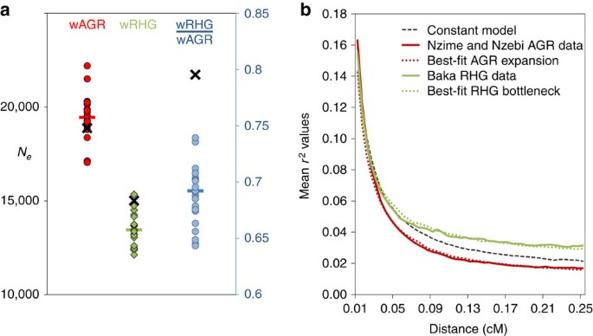Figure 4: Estimates of effective population sizes of Western RHG and AGR populations. (a) Recombination-based estimates of the effective population size of Baka RHG and Nzime/Nzebi AGR.Neestimates were obtained from the comparison of the inferred population-based and deCODE pedigree-based recombination maps. Each point represents an autosome. The horizontal bar represents the mean ofNefor the 22 autosomes, and a cross represents the X chromosome. Blue circles and right axis represent the ratio ofNeof RHG and AGR. (b) Demographic scenarios best-fitting observed LD decay in Baka RHG and Nzime/Nzebi AGR. A bottleneck model starting 16,000 YBP with 75% intensity best fitted LD decay in RHG, while an expansion starting 10,000 YBP with 20-times intensity was obtained for AGR. 2 ; Supplementary Table 4 ). AGR-to-RHG admixture rate estimates were thus on average 8.8 times larger than RHG-to-AGR estimates, supporting the occurrence of asymmetrical admixture from AGR to RHG populations. Figure 2: Admixture LD in RHG and AGR populations. Admixture LD signals were detected with ALDER, using the one-reference mode with 363,088 SNPs in 481 sub-Saharan Africans. Lines represent fitted exponential curves for significant AGR-to-RHG admixture signals. Results for all possible pairs are reported in Supplementary Table 4 . The AGR and RHG pairs plotted here correspond to populations that are known to interact today. If the corresponding AGR population was not sampled, or if a long-range LD correlation was observed between the two populations, the genetically closest AGR population was selected. Full size image Furthermore, our comparison of ancestry proportions on the X chromosome and the autosomes in AGR and some RHG populations, and a large body of studies based on uniparentally inherited markers [18] , [38] , [39] , suggest that during the admixture process there has been preferential mating of AGR males with RHG females ( Supplementary Note 2 , Supplementary Fig. 7 , Supplementary Tables 5 and 6 ). This is consistent with the present-day mating patterns of these communities; RHG women marry both RHG and AGR men—although the latter scenario is comparatively rare—while RHG men marry almost exclusively RHG women [7] , [8] , [10] , [35] , [40] . Our analyses also revealed, however, more balanced patterns in Baka and Batwa RHG, highlighting the heterogeneity and complexity of the admixture histories of RHG populations, and the need to perform extensive simulation studies to better understand the observed patterns. Recent onset of admixture in RHG populations To date the onset of admixture between RHG and AGR, we first used the number of ancestry blocks obtained from HAPMIX [41] but remarked that our results were highly sensitive to prior parameter values ( Supplementary Note 3 , Supplementary Figs 8 and 9 ). We thus instead used the ALDER approach [36] , [37] and fitted an exponential curve to the observed curves of admixture LD decay in RHG populations ( Fig. 2 ). Estimated times were more recent than 900 YBP in all RHG populations (mean: 437 YBP, Supplementary Table 7 ), much later than the 3,000–5,000 YBP expected if admixture had started at the initial phases of the spread of farming in these regions. Furthermore, time estimates varied substantially among RHG populations, ranging from 141 YBP (±s.e. of 29 YBP) in Bezan Western RHG to 886±55 YBP in Biaka Western RHG, revealing again considerable differences in the admixture history of these populations. Given the geographical proximity and long-term socio-economic interactions of RHG and AGR communities [7] , [8] , [15] , [42] , we reasoned that a model of continuous admixture may be more realistic than the single-pulse admixture model assumed by ALDER [37] , which might bias our time estimates downwards. Both the weak fitting of exponential curves with observed admixture LD curves ( Fig. 2 ) and the dependence of time estimates with the admixture LD starting point ( Supplementary Table 7 ) suggest that the single-pulse model is indeed less likely in RHG. On the other hand, when using equations relating the within-population variance of ancestry proportions to the time of admixture [43] , we found that the high variance of AGR ancestry proportions observed in most RHG populations ( Fig. 1 ; Table 1 ) was compatible with a single-pulse admixture event occurring only ~150 YBP, that is, approximately four times later than was estimated based on admixture LD decay ( Supplementary Table 7 ). Such a discrepancy between time estimates suggests that, in addition to the admixture occurring during or before the time period estimated by ALDER, recent admixture between RHG and AGR in the last generations has also occurred. We next tested the extent to which such recent, ongoing admixture has biased downwards ALDER time estimates, which correspond to a time weighted by admixture rates at each generation [37] . To do so, we re-estimated times by excluding the most highly admixed RHG individuals, that is, those who may have admixed during the last generations. Our estimations remained largely unchanged (mean: 466 YBP; maximum: 844±82 YBP; Supplementary Fig. 10 , Supplementary Table 8 ), indicating that the impact of recent admixture on ALDER estimates is negligible. Most importantly, under a model of continuous admixture with a constant rate, ALDER estimates would, at most, increase by twofold [37] . Time estimates averaged across RHG populations would thus be of 926 YBP, with a maximum of ~1,852 YBP in the Biaka (that is, twice the earliest time of admixture obtained, 844+82 YBP), still a few thousand years after the first farming communities encountered local hunter-gatherer groups. Reduced effective population sizes of RHG To explore further the demographic history of RHG and AGR groups, we focused on their population sizes and mating patterns in the past, by first examining the levels of homozygosity of their genomes. The extent of genomic runs of homozygosity (ROH) can record variation in consanguinity and cultural endogamy as well as effective population size. Specifically, consanguinity creates unexpectedly long ROH, while a low effective population size ( N e ) generally increases both number and length of ROH [22] , [44] . The number and length of ROH in RHG and AGR populations were summarized by the cumulative sum of ROH per genome (cROH). The population mean of cROH was higher in RHG (93.1–156.2 cM) than in AGR (59.4–84.0 cM), with the exception of both Bongo Western RHG groups (72.5 and 65.5 cM; Fig. 3a ; Supplementary Figs 11 and 12a ). The low cROH observed in the Bongo probably reflects their extensive admixture with neighbouring villagers. Consistent with this, cROH and RHG ancestry proportions were significantly positively correlated in most RHG populations (Pearson’s r =0.58, P <2.2 × 10 −16 ; Supplementary Fig. 12b ). Batwa Eastern RHG presented not only the highest cROH but also the highest proportion of long ROH of all populations: 4.0% of Batwa ROH were longer than 10 cM, while 1.2 and 0.3% of ROH met this criterion in the remaining RHG and AGR populations, respectively ( Supplementary Fig. 12a ). This suggests that consanguinity has increased further the levels of homozygosity observed in the Batwa. Altogether, our findings suggest lower N e and higher endogamy in RHG, with respect to AGR populations. Figure 3: Lower effective population sizes of RHG with respect to AGR populations. ( a ) Patterns of runs of homozygosity (ROH) in RHG and AGR populations. Cumulative ROH (cROH) is reported per population, against the total number of observed ROH. Population colour codes are reported in b . ( b ) LD decay with genetic distance in RHG and AGR populations. Pairwise r 2 values were obtained using Haploview, calculated between ~350,000 SNPs with minor allele frequency>5% in each population and averaged across 10 random samplings of 13 samples per population. On average, ~28 million values were obtained per population. Full size image We next interrogated another independent aspect of the data—the rate of LD decay with genetic distance—which is known to vary with N e as well as recombination rate [45] . We observed systematically slower rates of LD decay in all RHG populations, particularly in Batwa Eastern RHG, when compared with AGR ( Fig. 3b ). Importantly, our results were obtained after excluding RHG samples with extreme cROH or AGR ancestry proportions. In light of this, the high rates of inbreeding or admixture with AGR populations alone cannot explain the high LD levels observed in RHG, and reflect instead a lower N e of RHG with respect to AGR. Notably, the higher LD levels observed in Batwa Eastern RHG with respect to other RHG populations suggest that this population has experienced more genetic drift. Altogether, both ROH and LD decay results clearly support a lower effective population size of all forest-dwelling hunter-gathering populations with respect to AGR. Demographic regimes differed before agriculture emerged To formally test the impact of the emergence of agriculture on the demography of RHG and AGR, we estimated their global N e and its fluctuation over time, using population recombination rate estimates and LD levels (Methods). We hypothesized that the groups of Baka Western RHG, and Nzime and Nzebi AGR of Cameroon and Gabon represent the best study model, because they live close to the postulated homeland of Bantu-speaking farmers [4] , [5] , [6] . Furthermore, each group displayed little internal structure ( Fig. 1 ; Supplementary Table 2 ), contained a similar, large number of samples (70 and 73 unrelated individuals, respectively), included trios and duos that are critical for phase reconstruction [46] and showed limited recent admixture with each other ( Fig. 1 ). We phased RHG and AGR separately using SHAPEIT [47] , and estimated the effective recombination rate ρ (with ρ =4 N e r for autosomes and ρ =3 N e r for the X chromosome [48] , [49] ) in each population, using LDhat [50] . As expected, ρ estimates were highly correlated between the two populations (log-transformed rates per kb: r =0.89, t -test P <0.0001, Supplementary Fig. 13 ). N e was then estimated by comparing the total ρ map length of RHG and AGR genomes with the pedigree-based deCODE recombination map [51] . For autosomes, N e estimates of Western RHG ( N e =13,442, (12,118–15,333)) were lower than those of AGR ( N e =19,537, (17,038–22,185)), yielding an RHG-to-AGR N e ratio of 0.69 ((0.64–0.74)), Fig. 4a ; Supplementary Fig. 14 ). These results clearly attest to a systematic difference in effective population size between RHG and AGR communities. Figure 4: Estimates of effective population sizes of Western RHG and AGR populations. ( a ) Recombination-based estimates of the effective population size of Baka RHG and Nzime/Nzebi AGR. N e estimates were obtained from the comparison of the inferred population-based and deCODE pedigree-based recombination maps. Each point represents an autosome. The horizontal bar represents the mean of N e for the 22 autosomes, and a cross represents the X chromosome. Blue circles and right axis represent the ratio of N e of RHG and AGR. ( b ) Demographic scenarios best-fitting observed LD decay in Baka RHG and Nzime/Nzebi AGR. A bottleneck model starting 16,000 YBP with 75% intensity best fitted LD decay in RHG, while an expansion starting 10,000 YBP with 20-times intensity was obtained for AGR. Full size image Interestingly, such a difference in population sizes was less pronounced for the X chromosome. While the N e of AGR estimated from the X chromosome ( N e =18,864) was slightly lower than that estimated from autosomes ( N e =19,537), the N e of RHG from the X chromosome ( N e =15,001) was higher than that from autosomes ( N e =13,442; Fig. 4a ). This yielded an X-to-autosome N e ratio of 1.12 for RHG and 0.97 for AGR ( Fig. 4a ). We then estimated the female-to-male breeding ratio ( β = N f / N m ) using recently derived equations based on ρ estimates [48] , [49] . We obtained a clearly higher breeding ratio in RHG with respect to AGR ( β =1.68 and 0.77, respectively), supporting a higher effective population size of RHG females with respect to males. Such a distorted breeding ratio can be explained neither by a more frequent practice of polygyny in RHG than in AGR (that is, the inverse is systematically observed [7] , [11] , [40] , [42] ), nor by gender-biased gene flow and historical differences in the variance of reproductive success between AGR and RHG ( Supplementary Note 4 ), leaving open a variety of causes that remain to be explored. The estimated 30% reduction in effective population size of Western RHG with respect to AGR suggests that historically the demography of these populations has differed extensively. To gain insight into the nature and tempo of these events, we investigated further their levels of LD at increasing genetic distances. It has been shown that LD decay captures information on temporal fluctuations of N e , with LD between distant markers reflecting recent fluctuations in N e while LD between close markers being more affected by ancient N e (ref. 52 ). However, an important limitation of this approximation is that it no longer holds when the population has undergone marked reductions in size (that is, bottlenecks) [53] . To circumvent this limitation, we compared observed LD levels with those obtained by one million coalescent simulations of entire genomes, assuming instantaneous expansions or bottlenecks in a calibrated isolation-with-migration scenario and considering SNP ascertainment bias (Methods). In RHG, the 2% of models that best fit the data were bottlenecks ( N e reduction of 65–80%) occurring 10,000–31,000 YBP, while those best fitting the data in AGR were expansions ( N e increase of 5–45 times) occurring 7,000–10,000 YBP ( Figs 4b and 5 ). Importantly, when assuming such bottleneck and expansion best-fit models, the harmonic mean of N e over time was 12,288 and 18,074 for Western RHG and AGR, respectively, in agreement with our estimations using the population recombination rate ( Fig. 4a ). 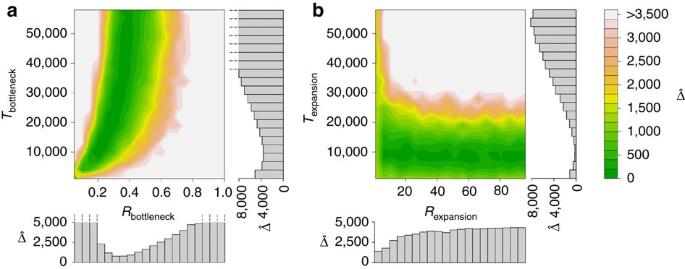Figure 5: Simulated models of a bottleneck and an expansion fitting the observed LD levels of Western RHG and AGR. (a) Fitting between the observed LD decay of Baka RHG and 400 models of bottleneck; (b) fitting between the observed LD decay in Nzime/Nzebi AGR and 400 models of expansion. TimesTare expressed in years. IntensitiesRof demographic events correspond to the ratio ofNeafter to before the corresponding event. Colours represent the distance Δ between the observed and the simulated LD decay curves (Methods). The smaller the Δ, the better the model fits the observed data. For convenience, all Δ distances that were higher than 3,500 were set to 3,500. Histograms represent the average of Δ for each parameter across all models. Figure 5: Simulated models of a bottleneck and an expansion fitting the observed LD levels of Western RHG and AGR. ( a ) Fitting between the observed LD decay of Baka RHG and 400 models of bottleneck; ( b ) fitting between the observed LD decay in Nzime/Nzebi AGR and 400 models of expansion. Times T are expressed in years. Intensities R of demographic events correspond to the ratio of N e after to before the corresponding event. Colours represent the distance Δ between the observed and the simulated LD decay curves (Methods). The smaller the Δ, the better the model fits the observed data. For convenience, all Δ distances that were higher than 3,500 were set to 3,500. Histograms represent the average of Δ for each parameter across all models. Full size image As recent admixture influences the levels of LD, we performed the same simulation study by removing the most highly admixed individuals from each population ( Fig. 1 ). The models best fitting the data were a slightly younger bottleneck in RHG ( N e reduction of 65–80%) occurring 7,000–22,000 YBP and an older expansion in AGR ( N e increase of 10–90 times) occurring 16,000–22,000 YBP ( Supplementary Fig. 15 ). To assess the robustness of these results, we replicated our approach 50 times on a subset of models, and confirmed that the 2% of models that initially best fit the data in RHG and AGR were indeed the best-fitting models in 100% of replicates (Methods). Furthermore, models in which bottlenecks and expansions occurred 4,000 YBP were rejected in 100% of these replications. Our results thus support the view that the difference in effective population sizes observed between Western RHG and AGR results from distinct demographic events that predate the first expansions of farming peoples in the Central African belt. Our genome-wide analysis has documented previously unknown levels of population structure among RHGs. Western RHG populations represent a weakly differentiated but structured genetic entity, consistent with their recent separation proposed to be triggered by the expansions of Bantu-speaking farmers [25] . Conversely, an unexpected degree of genetic differentiation was observed between the two Eastern RHG populations, given their geographic distance. The similar admixture rates of Batwa and Mbuti RHG with non-RHG populations of Central and Eastern Africa ( Supplementary Note 1 ), together with their elevated levels of homozygosity and LD, suggest that genetic isolation, strong drift in populations of small effective sizes and/or endogamy have collectively contributed to their differentiation. More generally, the varying degrees of population structure and farmer ancestry detected among the different Western and Eastern RHG populations emphasize the complexity and specificity of their past history, as well as the interactions that each of them have maintained with the neighbouring farmers. Despite this observed heterogeneity, two major, novel observations emerge from our study. First, we show that the bulk of the admixture between various groups of RHG and neighbouring AGR took place only recently, within the past ~1,000 years. This indicates that the earliest phase of the diffusion of an agriculture-based lifestyle, where an avant-garde of farming communities in the Western (c. 3,000–5,000 YBP) and Eastern (c. 2,500–3,000 YBP) equatorial rainforest [3] , [6] , [15] , [54] promoted early socio-economic and cultural interactions with local RHG [2] , [3] , [7] , [8] , [11] , [15] , [16] , [17] , [18] , [19] , was not accompanied by immediate, extensive genetic exchanges. Our results suggest instead that admixture started extensively at a later stage, well after the introduction of iron tools and plant cultivation and the subsequent rise of territorial chiefdoms, profoundly transforming the interactions between the two communities [15] , [42] . This slow, two-phased process of interactions greatly differs from that recently documented in Southern Africa [55] , where it appears to have been more rapid and different in its outcome. Indeed, as soon as agro-pastoralists reached the Kalahari desert ~1,200 YBP [3] , [56] , [57] , their encounters with local Khoisan hunter-gatherers resulted in immediate genetic exchanges [55] but not in language shifts, as Khoisan groups have retained their own non-Bantu languages with click consonants. Conversely, the long period of intimate interactions between RHG and AGR in Central Africa, owing to their socio-economic and ecological interdependence [42] , was accompanied by complete language shifts in all RHG groups [33] . We suggest that such complex interactions have been, however, also socially controlled, as attested by the strong cultural barriers against intermarriages currently observed [7] , [8] , [10] , [35] , [40] , preventing for a long period of time extensive genetic exchanges between the two communities. Second, we find that the demographic regimes of contemporary RHG and AGR living close to the epicentre of the expansions of Bantu-speaking peoples were already distinct before the emergence of agriculture. The signal of reduced effective population size of RHG populations detected here has previously been observed in some other RHG groups, consistent with the occurrence of past bottlenecks [21] , [22] , [23] , [24] , [39] . Our study, however, provides with novel information concerning the intensity and time depth of such demographic events. We show that the effective population size of RHG is ~30% lower than that of AGR, at least in Western Central Africa, as a result of a bottleneck and an expansion occurring earlier than 7,000 YBP in the ancestors of RHG and AGR, respectively. Previous studies have indeed estimated that the ancestors of African farmers started to expand ~10,000–30,000 YBP using other aspects of the data such as the allele frequency spectrum [58] , [59] , [60] . Our analyses of LD levels thus reinforce these findings, and support the notion that the expansions of Bantu-speaking peoples 3,000–5,000 YBP are not sufficient to explain the signal of population growth observed in present-day AGR. Future studies based on full sequencing data from thousands of individuals, allowing the detection of low-frequency variants, should enable to evaluate how such recent expansions have also left their traces on the genomes of African populations. To conclude, our study indicates that the ancestors of contemporary African farmers were already demographically successful before agriculture, possibly facilitating their transition to a food-producing lifestyle and its subsequent transmission to the rest of the continent. Our data also support the view that, while the first expansions of Bantu-speaking farmers set the ground for social, economic and cultural interactions between them and forest-dwelling hunter-gatherers, they did not directly trigger immediate, extensive genetic exchanges between both communities. Population samples A total of 327 individuals representing eight different human populations of Central Africa were included in this study. Our sample of Western Central Africans included 35 unrelated Baka RHG as well as 16 trios, and 27 unrelated Nzime AGR as well as 16 trios from Cameroon; 20 unrelated Baka RHG and 20 unrelated Nzebi AGR from Gabon; 24 unrelated Bongo RHG from East Gabon; and 25 unrelated Bongo RHG from south Gabon. Our sample of Eastern Central Africans included 40 unrelated Batwa RHG and 40 unrelated Bakiga AGR from Uganda. Informed consent was obtained from all participants and from both parents of any participants aged under 18. This study obtained ethical approval from the Institutional Review Boards of Institut Pasteur, France (RBM 2008-06 and 2011-54/IRB/2), Makerere University, Uganda (IRB 2009-137) and University of Chicago, USA (16986A). Genome-wide genotyping The 327 samples were genotyped on the Illumina HumanOmni1-Quad genotyping array (Illumina, San Diego, USA) at the genotyping platform of the Institut Pasteur, Paris, France. Genotypes of 1,048,713 SNPs were called in all samples using the Illumina Genome Studio v2010. SNPs were excluded if they had a GenTrain score <0.35, a call rate <95% or if they were insertion-deletions, unmapped on Human Genome build 37, duplicated or located on several chromosomes. In total, 930,134 autosomal and X-linked SNPs passed quality control filters ( Supplementary Fig. 1 ). For these SNPs, the average genotype concordance rate across seven pairs of duplicated samples was 99.91%. Genotype calling of uniparentally inherited SNPs was performed manually by visual inspection of genotype clusters in Genome Studio. One hundred and seventy four Y-linked SNPs and 12 mitochondrial DNA SNPs were polymorphic in our sample. Sample exclusion Of the 327 genotyped samples, 9 individuals were excluded because of a call rate <95%. Relatedness among our samples was evaluated by estimating the relatedness coefficient of all possible pairs of samples, using the pairwise correlation coefficient implemented in smartrel, corrected for the top eigenvalues obtained using the EIGENSTRAT program [31] . We consistently obtained a coefficient of ~0.5 for most of parent–offspring pairs (average: 0.48, s.d. : 0.007). However, five parent–offspring pairs presented unexpectedly low coefficients (<0.10). Using PLINK [61] , we obtained a rate of Mendelian inconsistencies >10% for the five corresponding trios, while this rate was <0.05% in all the other complete trios. In all subsequent analyses, the five trios were considered as duos or as unrelated samples. We also observed cryptic relatedness among our samples: 23 pairs of samples exceeded a correlation coefficient of 0.3, so 23 individuals were excluded, including 15 RHG and 8 AGR individuals. Two hundred and ninety-five individuals were retained for subsequent analyses, including 216 unrelated individuals, 21 complete trios and 8 duos, giving a total of 266 unrelated samples ( Supplementary Fig. 1 ). Data from previous studies We merged our genotyping data for 930,134 SNPs in 295 individuals with data for 221 additional samples, retrieved from previous studies [26] , [29] . Namely, we selected 96 individuals from five human genome diversity panel (HGDP) sub-Saharan African populations genotyped for 636,647 SNPs [29] (that is, Biaka RHG of CAR, Mbuti RHG of Democratic Republic of Congo, Yoruba AGR of Nigeria, Mandenka AGR of Senegal and Bantu-speaking AGR of Kenya, Supplementary Table 1 ), and 125 individuals from six populations of Cameroon genotyped for 1,083,209 SNPs [26] (that is, Baka RHG, Bakola RHG, Bezan RHG, Lemande AGR, Ngumba AGR and Tikar AGR, Supplementary Table 1 ; dbGaP study accession: phs000449.v2.p1). We restricted the three data sets to the SNPs that were genotyped in all, yielding a total of 363,088 polymorphic SNPs in 516 individuals. No relatedness or population differentiation was detected between the Baka RHG of Cameroon of this study and those retrieved from a previous study [26] ; the two populations were thus considered as a single population in all subsequent analyses. Runs of homozygosity We searched for ROH within the genome of the selected 516 African individuals. To minimize the bias introduced by SNP ascertainment, we restricted this analysis to 165,702 SNPs whose population frequency was higher than 5% in every population. We used the sliding window approach implemented in PLINK [61] . The whole genome of each sample was explored by a sliding window of 50 SNPs. If the 50 SNPs were homozygous in the individual considered, the window was considered as homozygous, with the possible exception of two heterozygous SNPs and allowing for five missing genotypes. ROH regions were defined as regions of at least 500 kb in which all SNPs were included in at least one homozygous window. Previous studies have used a minimum ROH length of 1 Mb (refs 62 , 63 ) to discern inbreeding from strong LD on homozygosity segments. However, recent studies focusing on the history of human populations [44] , and particularly on sub-Saharan Africans who present lower levels of LD [22] , have privileged a minimum ROH length of 500 kb. We also specified that ROH regions must present a SNP density of at least one SNP every 50 kb. The number, length distribution and the cumulative length of ROH regions (cROH) in each individual were then analysed. Six individuals presented unusual cROH, that is, four s.d. higher than the average of his/her population of origin, which was considered as evidence of recent inbreeding. As methods to infer genetic ancestry assume random mating among individuals, we excluded these six samples from subsequent analyses. Our final filtered data set thus included a total of 481 unrelated samples, that is, 260 unrelated samples studied here and 221 samples from previous studies [26] , [29] . Population structure and differentiation To gain insight into the population structure of our samples, the unsupervised clustering algorithm Admixture [30] was used on our filtered data set of 481 unrelated individuals, for 310,883 SNPs, after pruning SNP pairs with r 2 >0.5 using PLINK [61] . Ten runs were performed for each K value, ranging from 2 to 15. K =3 runs produced the lowest mean cross-validation error rate ( Supplementary Fig. 3 ), that is, the value of K for which the model has best predictive accuracy [30] . In all subsequent analyses that were restricted to the least admixed samples, we excluded from each population the 25% of samples with the highest admixture proportions at K =3. The PC analysis implemented in EIGENSTRAT [31] was performed on the same data set. Genetic differentiation between populations was computed for all autosomal, X-linked, Y-linked and mitochondrial DNA SNPs using the analysis of molecular variance implemented in Arlequin v.3 (ref. 64 ). Haplotype-based population structure We compared the results obtained with EIGENSTRAT, which assumes independence among SNPs, with the results of ChromoPainter/fineSTRUCTURE, a recent method that infers population structure based on haplotype similarity [65] . Our 289 samples genotyped for 930,134 SNPs were phased and missing data were imputed using SHAPEIT v.2 (ref. 47 ), accounting for trios and duos. The genetic map was obtained from the HapMap phase 2 recombination map [66] , after interpolating by local linear regression the SNPs that were absent from the map. We specified a N e of 15,000 individuals ( N e estimated from 10 expectation-maximization iterations was ~16,000). The Monte Carlo Markov chain of fineSTRUCTURE was made of 10 million iterations as burn-in, 10 million iterations as runtime and with sampling every 1,000 iterations. Tree building was performed with default parameters ( Supplementary Fig. 4 ). Inferred geographic location of Baka To test the hypothesis that the Baka originate from the CAR, where they might have acquired their Ubangian language and formed a unique group with the Biaka, we considered the geographic location of the Baka unknown and deduced expected geographic distances between Baka and all other RHG populations from both the observed F ST values and the regression equation of the isolation-by-distance relationship among all RHG populations except the Baka ( Supplementary Fig. 5b ). The inferred geographic location of the Baka was then deduced by calculating for 17,000 geographic coordinates the difference between geographic distances to the other RHG populations implied by the tested coordinates and those expected under isolation-by-distance ( Supplementary Fig. 5c ). The coordinates with the lowest differences (green colour grade in Supplementary Fig. 5d ) were considered as the most parsimonious inferred geographic locations of the Baka. The map was obtained with the ggmap R package. Admixture LD To formally test for admixture and to estimate time since admixture between RHG and AGR, we used ALDER [37] . Four hundred and eighty-one individuals and 363,088 SNPs were considered for this analysis. All possible pairs of populations were tested using the one-reference mode ( Supplementary Table 4 ), given the absence in our sample of a non-admixed RHG reference population. We then checked the consistency of the single-pulse model of admixture assumed by the program by calculating the distance between observed data and exponential fitted curves (that is, the mean-squared difference of observed and expected values), and by calculating the slope of a linear function relating the estimated time since admixture and d 0 , the first bin of genetic distance considered for time estimation. If admixture rates have fluctuated in time, the admixture LD decay curve will be composed of a series of curves with different decay rates [37] , and the time estimated by ALDER will depend on d 0 . LD decay We computed the r 2 LD statistic between every possible pair of SNPs in a 1-Mb sliding window using Haploview [67] . The 25% of most highly admixed samples and the 10% presenting the highest cROH were discarded from the analysis. As the r 2 statistic is sensitive to sample size, we randomly selected 13 individuals in each population sample, corresponding to the lowest sample size studied (after excluding Bantu-speaking AGR of Kenya) and repeated resampling and r 2 calculations ten times. To avoid any bias introduced by SNP ascertainment, we restricted this analysis to ~350,000 SNPs whose population frequency was higher than 5% in every population subsample. About 28 million r 2 values were obtained per population in each of the 10 replicates. Genetic distances between every pair of SNPs were retrieved from the HapMap phase 2 recombination map. All pairwise r 2 values were then grouped into 50 bins of increasing genetic distance and averaged per bin. Population recombination rate and N e estimation 70 Baka Western RHG and 73 Nzime/Nzebi Western AGR were phased separately using SHAPEIT v.2 (ref. 47 ), accounting for trios and duos. We then used the Markov Chain Monte Carlo method implemented in LDhat v.2.1 (ref. 50 ) to estimate the population recombination map. All autosomes—and the X chromosome in females and males separately—were explored by a sliding window of 2,000 SNPs, with an overlap of 500 SNPs between contiguous windows. Five million iterations were performed per window, 500,000 samples were removed as burn-in and sampling was done every 5,000 iterations. In overlapping segments, rate estimates from the last 250 SNPs of the 5′-region window and the first 250 SNPs from the 3′-region window were removed. We estimated the effective population sizes N e of Western RHG and AGR from the comparison of the genetic maps estimated here and the pedigree-based, sex-averaged, deCODE genetic map [51] . Demographic inference based on LD decay We estimated LD decay as described above, but restricted our population sample to our two model populations: Baka Western RHG and Nzime/Nzebi Western AGR. To avoid any bias introduced by SNP ascertainment, we restricted this analysis to SNPs whose population frequency was higher than 5% in both populations. To determine the demographic models that best explain observed LD decay in Western RHG and AGR, we performed coalescent simulations using the program MaCS [68] . We simulated two populations under an isolation-with-migration model, with sample sizes of 70 and 73 diploid individuals ( Figs 4b and 5 ) or 55 and 55 diploid individuals ( Supplementary Fig. 15 ). The ancestral population size, the time of divergence and the migration rate between the two populations were sampled from posterior distributions of parameter estimates, obtained previously for the same populations using autosomal resequencing data [23] . We verified that the sampled values of these three parameters produced an F ST value between simulated populations (from 0.01 to 0.04, depending on the model) compatible with that observed ( F ST =0.023, Supplementary Table 2 ). We simulated two different demographic models, that is, an instantaneous expansion with intensities ranging from 1 to 100, occurring 1,000 to 60,000 years ago, and an instantaneous bottleneck with intensities ranging from 0.05 to 1, occurring 1,000 to 60,000 years ago. Intensity and time parameters could take 20 values each, resulting in 400 possible parameter sets for each model. We performed 1,000 simulations of 2-Mb regions per parameter set, and specified for each simulated region a recombination map that was drawn from the HapMap phase 2 recombination map, to match the recombination hotspot structure of the human genome. To simulate SNP ascertainment bias, we sampled simulated SNPs to match the observed site frequency spectrum of our genotyping data set, and then randomly drew SNPs to match the SNP density of our data set. We computed all possible pairwise r 2 values for each simulated 2-Mb region using Haploview [67] , retrieved genetic distances between SNP pairs according to the recombination map specified in MaCS and merged r 2 distributions of all simulations, binned by genetic distance. For each parameter set, we ultimately obtained a LD decay curve based on 30–40 million r 2 values. To identify the model best fitting the observed data, we calculated, for each simulated LD decay curve, a distance metrics Δ model with the observed LD decay curve where Δ model corresponds to the mean χ 2 statistics comparing n =50 observed and simulated r 2 values along the two curves. To test the accuracy of our method, we resimulated 50 times the 2% best-fitting models (that is, eight models) obtained for Western RHG and AGR, together with a couple of models that were between the top 2% and 5% best models. Interestingly, the initial 2% best-fitting models consistently better fit the data than all others, in 100% of replications. Furthermore, among this 2%, the two initially best-fitting models were once again identified as the best-fitting ones in 100 and 60% of replicates, for the RHG bottleneck and the AGR expansion, respectively. To test the hypothesis that Bantu expansions were responsible or not for the bottleneck and expansion signals obtained in RHG and AGR, respectively, we also resimulated 50 times the best-fitting bottleneck or expansion models with fixed onset at T =4,000 YBP, which were not initially found among the 2% of best-fitting scenarios. We showed that such scenarios—that is, a bottleneck and an expansion occurring T =4,000 YBP—were consistently rejected in 100% of the replications. Accession codes: Genotype data for the Central African rainforest hunter-gatherers and neighbouring agriculturalists have been deposited in the European Genome-phenome Archive under accession code EGAS00001000605. How to cite this article: Patin, E. et al. The impact of agricultural emergence on the genetic history of African rainforest hunter-gatherers and agriculturalists. Nat. Commun. 5:3163 doi: 10.1038/ncomms4163 (2014).